Electrically controlled one-way photon flow in plasmonic nanostructures Photonics is frequently regarded as a potential pathway for substituting current solid-state electronics and as a promise for higher-speed all-optical computing. The fundamental challenges facing nanophotonics and electronics of the future are nanoscale on-chip integration of electronics and photonics with an efficient electric field tuning of light propagation, dynamic access to the light sources and material parameters of the system, as well as isolation of optical signals analogous to that in electronics. Here we suggest a paradigm for a monolithically integrated electronic control over the light propagation in nanoscale plasmonic waveguides. We theoretically demonstrate that magnetic field induced by the direct electric current flowing in metallic constituents of plasmonic nanostructures alters the material parameters and thus the optical signal flow. We use this principle for the design of an electrically controlled subwavelength optical isolator. Recent progress in silicon photonics, plasmonics and graphene has allowed miniaturization of basic elements of integrated optics well beyond the light diffraction limit [1] , [2] , [3] , [4] . Many important electromagnetic analogs of electronic circuit elements have been suggested and developed lately, including interconnects [2] , optical analogues for capacitors and inductors (the so-called optical metatronic elements [5] ), nonlinear optical diodes [6] and isolators [7] , [8] . Nonetheless, the functionality of an on-chip signal processing optical network crucially depends on its compatibility with electronics, as well as on its tunability with external stimuli [9] , [10] , [11] , [12] . However, the direct action of an electric field effect at high frequencies (that is, upper terahertz, telecom and visible wavelength ranges) associated primarily with the change of material parameters ( ε or μ ) is weak and is practically not used in applications [13] , [14] . (Note that the electro-optical manipulation is successfully implemented at microwave and terahertz frequencies, particularly in two-dimensional plasmonic systems. [3] , [4] ). On the other hand, an electric direct current (DC) in a conductor, for example, a piece of wire, always creates a DC magnetic induction around the conductor. As we shall show in this work, it is this induction field that can be employed for an efficient tuning and control of electromagnetic waves guided along the wire. Light propagation in a magnetized medium has attracted interest for a long time, following the discovery of nonreciprocal polarization rotation by Michael Faraday [15] . However, interest in magneto-optical activity has been resurrected in recent years due to its ability to efficiently tune light–matter interaction in nanoscale optical systems [11] , [16] , [17] and to break the time-reversal symmetry [18] , [19] —a property vital for optical isolation [20] , [21] . Here we suggest a concept for merging electronics with nonreciprocal photonics at the nanoscale, that is, an electric tuning and control over electromagnetic fields within the fraction of a wavelength. We predict that material magnetization induced by the electric current in a wire can be used to manipulate propagation and isolation of electromagnetic fields by breaking the symmetry in wave excitation and propagation. Electrically controlled nonreciprocal plasmonics Consider a single metallic cylindrical nanowire with circular cross-section of radius R and with a DC I flowing in it, as shown schematically in Fig. 1a . A circulating magnetic induction B is induced outside and inside the wire, which for an infinitely long straight wire is given by the simple Biot–Savart formula [13] : inside the wire and outside it, where μ 0 is the vacuum permeability, ρ is the radial coordinate. The typical profile of the azimuthally symmetric field B is shown in Fig. 1b . The magnetic induction B acts on the wire itself and on the surrounding dielectric medium, generating magneto-optical response (when the dielectric is appropriately chosen), which can be triggered and controlled by the electric current I . 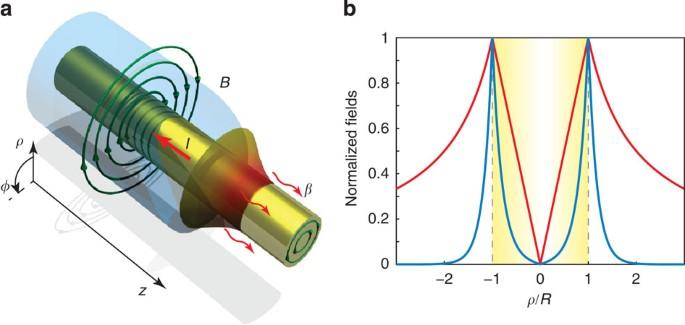Figure 1: Concept of a monolithically integrated electrically controlled plasmonic waveguide. (a) Geometry of the problem. Electric current flowing in a nanowire induces a circulating magnetic field that breaks the symmetry of surface plasmon polariton (SPP) propagation along the wire due to the presence of magneto-optical materials. Fundamental, azimuthally symmetric plasmonic mode is also shown. (b) Normalized radial profiles of electrically induced magnetic inductionB(red curve) and ofHϕcomponent of the fundamental SPP mode (blue curve) along the nanowire. In this case the electrodynamic properties of the media can, in general, be described by a dielectric permittivity tensor: Figure 1: Concept of a monolithically integrated electrically controlled plasmonic waveguide. ( a ) Geometry of the problem. Electric current flowing in a nanowire induces a circulating magnetic field that breaks the symmetry of surface plasmon polariton (SPP) propagation along the wire due to the presence of magneto-optical materials. Fundamental, azimuthally symmetric plasmonic mode is also shown. ( b ) Normalized radial profiles of electrically induced magnetic induction B (red curve) and of H ϕ component of the fundamental SPP mode (blue curve) along the nanowire. Full size image Here α is the off-diagonal component of the permittivity tensor responsible for the strength of the magneto-optical activity, ε ⊥ and ε mo are the relative dieletric permittivity tensor components along the magnetic bias and normal to it, respectively; the tensor should be considered in a cylindrical ( ρ , φ , z ) coordinate system. Note also, that the components of the tensor depend on the local intensity of the magnetic induction (Methods). At the same time the nanowire can serve as a plasmonic waveguide for surface plasmon-polaritons (SPP) [22] at optical frequencies, which are highly confined near the nanowire interface and are sensitive to the dielectric permittivity of the surrounding medium in the proximity of the wire. Figure 1b shows the typical profile of the SPP field. Clearly, the strongest magnetic action induced by the electric current I is at the interface of the wire with the surrounding medium, where the plasmonic field is also at its maximum, and, hence, a strong influence on SPP propagation and excitation even at moderate electric currents is expected, as will be discussed shortly. Such a natural compatibility and proximity between electric current and the photon field does not require bulky magnets (or electromagnetic systems), providing a platform for light weight, on-chip integrated, monolithic electro-optical nanosystems. Plamonic nanowire coated with a magneto-optical medium To demonstrate our concept we consider propagation of fundamental SPP mode, that is, azimuthally symmetric plasmons along gold nanowire with a 100-nm radius embedded into a bismuth iron garnet, a commonly available magneto-optical material, which saturates at B =150 mT (ref. 23 ). Such intensity of the magnetic induction B at the surface of the wire can be achieved with I =75 mA (the issues regarding the high value of current and its consequences and remedies are studied in the Supplementary Figs 2–4 , and Supplementary Notes 1–3 ). 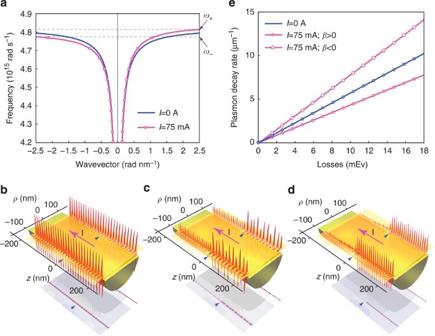Figure 2: Electric current control of plasmon propagation in a gold nanowire surrounded by a magneto-active dielectric. (a) Dispersion of plasmons with and without current flow in the wire in a lossless regime (that is, electron collision frequency,γ→0). Symmetry breaking in the dispersion relations is clearly seen. (Here points correspond to the exact solutions of the plasmon dispersion, whereas curves denote the solution of approximate dispersion relation, seeSupplementary Note 1). (b–d) Numerical simulations showing cross-sections of theHϕcomponent of the surface plasmon-polariton mode in several characteristic regimes of operation (here losses in the wire are neglected to display the concept): (b) plasmon excitation in an electrically neutral system (that is,I=0 A) atω=4.76 × 1015rad s−1clearly demonstrating symmetry in SPP propagation and excitation in ±zdirections; (c) excitation of plasmons forI=75 mA andω=4.76 × 1015rad s−1, at this frequency plasmons can propagate in both directions; however, the electric current in the wire breaks the symmetry of plasmon excitation and propagation; and (d) excitation of plasmons in a one-way regime atω=4.78 × 1015rad s−1andI=75 mA shows that plasmons are excited only in +zdirection. (e) Plasmon decay rate versus losses in the wire (that is, electron collision frequencyγ) with and without electric current in the wire calculated forω=4.75 × 1015rad s−1. Figure 2a shows the dispersion of SPP wave along the wire with and without the electric current in the wire (the dispersion relation and its analysis can be found in the Supplementary Note 1 ). When there is no current flow, the dispersion of plasmons propagating in + z and − z directions is symmetric and the system is reciprocal. For non-zero current in the wire the electrically induced magneto-optical activity in the bismuth iron garnet alters the dispersion of plasmons propagating in ± z directions. In particular, a break of symmetry in the dispersion of plasmons propagating in positive and negative directions along the wire occurs. In this case the waveguide becomes nonreciprocal, that is, β + ( ω )≠ β _( ω ) (similar dynamics was found for planar plasmonic waveguides [8] , [19] , [24] ). Furthermore, the SPP resonance frequencies corresponding to the condition β ± →∞ (that is, ε m =−( ε mo ± α ), ε m is the metal permittivity, see Methods), split for + z and − z directions of propagation: . In the range of frequencies ω sp ( β _)< ω < ω sp ( β + ) for an idealistic lossless system, only one-way SPP propagating in + z direction exists (we assume here that the current I propagates in − z direction; reversal of direction of current flow implies reversal of the symmetry breaking). The latter regime can be used for optical isolation. Figure 2: Electric current control of plasmon propagation in a gold nanowire surrounded by a magneto-active dielectric. ( a ) Dispersion of plasmons with and without current flow in the wire in a lossless regime (that is, electron collision frequency, γ →0). Symmetry breaking in the dispersion relations is clearly seen. (Here points correspond to the exact solutions of the plasmon dispersion, whereas curves denote the solution of approximate dispersion relation, see Supplementary Note 1 ). ( b – d ) Numerical simulations showing cross-sections of the H ϕ component of the surface plasmon-polariton mode in several characteristic regimes of operation (here losses in the wire are neglected to display the concept): ( b ) plasmon excitation in an electrically neutral system (that is, I =0 A) at ω =4.76 × 10 15 rad s −1 clearly demonstrating symmetry in SPP propagation and excitation in ± z directions; ( c ) excitation of plasmons for I =75 mA and ω =4.76 × 10 15 rad s −1 , at this frequency plasmons can propagate in both directions; however, the electric current in the wire breaks the symmetry of plasmon excitation and propagation; and ( d ) excitation of plasmons in a one-way regime at ω =4.78 × 10 15 rad s −1 and I =75 mA shows that plasmons are excited only in + z direction. ( e ) Plasmon decay rate versus losses in the wire (that is, electron collision frequency γ ) with and without electric current in the wire calculated for ω =4.75 × 10 15 rad s −1 . Full size image Figure 2b–d show numerical simulations of SPP excitation and propagation along the nanowire for several characteristic regimes of operation. As is predicted by the SPP dispersion relation, plasmon excitation and propagation is symmetric in the absence of the electric current in the nanowire, Fig. 2b . When the electric current in the wire is on, nonreciprocal symmetry breaking occurs ( Fig. 2c ), which is stronger as the operating frequency approaching the SPP resonance, ω ( β _), see also the SPP dispersion in Fig. 2a . In the regime of one-way propagation, that is, for operating frequencies in the range [ ω ( β _), ω ( β + )], Fig. 2d , plasmons can propagate only in the + z direction, and practically nothing is excited in the − z direction. Losses have an important role in plasmonics, reducing the performance of many of plasmonic devices significantly [22] . In Fig. 2e , numerically calculated distance of SPP propagation versus the electron collision frequency in the gold wire, that is, losses, is plotted. In the presence of the electric current in the nanowire plasmon attenuation in + z and − z directions differs significantly: plasmons propagating in the − z direction are strongly suppressed, whereas the decay rate for plasmons in + z is even weaker than that for plasmons in electrically and magnetically neutral system. Such a significant symmetry breaking in the plasmon propagation and their attenuation (see also Fig. 2c ) can serve as a platform for efficient electrically controlled on-chip subwavelength nonreciprocal devices. Magneto-optical activity in the conducting wire Generally magneto-optical activity is observed not only in the magneto-optical dielectrics, but also in transition metals, such as iron, nickel, cobalt and in conductors near the cyclotron frequency ( ω c = eB / m *, where e and m * are the electric charge and the effective mass of the electron in the conductor). The concept of electrically controlled symmetry breaking and nonreciprocity discussed earlier can be extended to these cases as well, assuming that the frequency of operation is close to the characteristic frequency of the magnetic resonance in the conductor, for example, cyclotron frequency. The latter can be achieved with the use of semiconductors with plasma frequency at THz frequencies or with corrugated metals supporting spoof plasmons ( Supplementary Fig. 2 and Supplementary Note 2 ). Consider, as an example, an indium arsenide (InAs) semiconductor wire 10 μm radius in a conventional dielectric background with permittivity ε d =6.25. Such a wire supports surface plasmon-polaritons in a terahertz frequency range. The dispersion of SPP propagating in ± z directions with and without electric current in the wire is shown in Fig. 3a,b . Below the SPP resonance, Fig. 3a , the plasmon dynamics is similar to that discussed earlier, see also Supplementary Fig. 1 and Supplementary Note 1 for more details. Above the SPP resonance, magnetically induced regimes of plasmon propagation emerge, Fig. 3b , that is, these regimes of plasmon propagation do not exist in an electrically neutral wire when the magneto-optical activity is zero [25] . They appear near the bulk plasma resonance of the magneto-active semiconductor core, and are associated with an effective metal-dielectric transitions in the presence of magneto-optical activity and emergence of the light-line in the semiconductor itself. Noticeably, corresponding regimes of plasmon-polariton propagation are one-way. Furthermore, the analysis of the dispersion relation shows that one of the dispersion branches corresponds to backward plasmonic waves, so that the directions of phase progression and energy propagation are opposite. 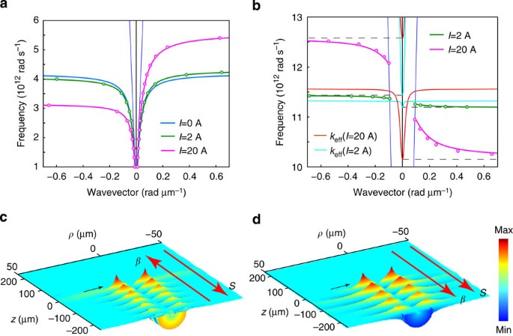Figure 3: Electronic tuning of a magneto-active semiconductor wire and control of surface plasmon-polariton propagation. (a) Plasmon dispersion below the surface plasmon-polariton resonance frequency for different levels of the electric current in the wire. (Note that such high values of electric current are chosen to demonstrate clearly the concept—the break of the symmetry is observed for smaller currents (≃0.1 A) as well. The possibility for enhancing symmetry breaking keeping electric current small is discussed in theSupplementary Notes 2 and 3). (b) Dispersion of guided surface wave around the bulk plasma frequency of the semiconductor core. Solid lines correspond to the light lines in the dielectric host (that is,). Dashed lines denote the range of plasmon existence with respect to the light-line of the magneto-active semiconductor corekeff. (Inaandb, points correspond to the exact solutions of the plasmon dispersion, whereas curves denote the solution of approximate dispersion relation, seeSupplementary Note 1). (c,d) Cross-sections of theHϕcomponent of the excited SPP field near the bulk plasma frequency of the semiconductor,ωp, in the presence of electric current in the wireI=20 A. (c) Belowωpatω=10.5 × 1012rad s−1, only one-way backward plasmonic mode is excited (that is, energy flow and phase propagation directions are opposite to each other). Atω=12.3 1012rad s−1, only plasmons propagating in −zdirection exist (d). Note that thezaxis is reversed for convenience. In all of the results shown here, loss in the semiconductor is neglected to display the concept. (For the detailed analysis of the losses and corresponding symmetry breaking, seeSupplementary Fig. 1andSupplementary Note 1). Figure 3c,d demonstrate the numerical simulation of the SPP excitation and propagation for both of the observed dispersion branches. Unidirectional excitation and backward wave propagation are clearly seen. Figure 3: Electronic tuning of a magneto-active semiconductor wire and control of surface plasmon-polariton propagation. ( a ) Plasmon dispersion below the surface plasmon-polariton resonance frequency for different levels of the electric current in the wire. (Note that such high values of electric current are chosen to demonstrate clearly the concept—the break of the symmetry is observed for smaller currents ( ≃ 0.1 A) as well. The possibility for enhancing symmetry breaking keeping electric current small is discussed in the Supplementary Notes 2 and 3 ). ( b ) Dispersion of guided surface wave around the bulk plasma frequency of the semiconductor core. Solid lines correspond to the light lines in the dielectric host (that is, ). Dashed lines denote the range of plasmon existence with respect to the light-line of the magneto-active semiconductor core k e ff . (In a and b , points correspond to the exact solutions of the plasmon dispersion, whereas curves denote the solution of approximate dispersion relation, see Supplementary Note 1 ). ( c , d ) Cross-sections of the H ϕ component of the excited SPP field near the bulk plasma frequency of the semiconductor, ω p , in the presence of electric current in the wire I =20 A. ( c ) Below ω p at ω =10.5 × 10 12 rad s −1 , only one-way backward plasmonic mode is excited (that is, energy flow and phase propagation directions are opposite to each other). At ω =12.3 10 12 rad s −1 , only plasmons propagating in − z direction exist ( d ). Note that the z axis is reversed for convenience. In all of the results shown here, loss in the semiconductor is neglected to display the concept. (For the detailed analysis of the losses and corresponding symmetry breaking, see Supplementary Fig. 1 and Supplementary Note 1 ). Full size image The concept we have introduced here can be employed for the design of next generation of monolithically integrated electrically tunable plasmonic waveguides and isolators. We note that the principles of electric field tuning developed in this work are not limited to a plasmonic waveguide problem. The proposed paradigm can be used in a wide range of problems and extended to design more complex systems, such as electric field tuning of the light scattering by plasmonic nanostructures [26] and electrically controlled Faraday rotation in plasmonic gratings [17] . Material parameters and numerical simulations Dispersions of surface plasmon-polaritons in the presence of electric current taking into account the radial variation of the magnetic field have been solved numerically with a shooting method. (For details, see Supplementary Note 1 ). Numerical simulations shown in Fig. 2b–d and Fig. 3c,d have been performed with the finite-element method commercially available in COMSOL Multiphysics environment. In our numerical simulations we have excited fundamental, azimuthally symmetric plasmons with a looped magnetic current. In an experiment setup, such plasmons may be excited by a radially polarized laser beams [27] or via mode transformation technique [28] . In our analysis, we have modeled both gold and indium arsenide with a Drude–Lorentz model: and , where ω p is the plasma frequency, γ is the effective electron collision frequency, responsible for the material loss, and ω c = eB / m * is the cyclotron frequency with e and m * being charge and effective mass of electron, respectively. For gold we have assumed ω c ≡0, since the magneto-optical activity in gold at optical frequencies is several orders of magnitude weaker than that in bismuth iron garnet; the values for the bulk plasma and electron collision frequencies in gold have been taken from ref. 29 . It is worth noting that, such a model for gold permittivity is not accurate at optical frequencies due to a strong influence of interband transitions, however, our concept is not limited to this specific material dispersion and one can easily take into account a more complex material response and more complicated structures. The parameters for indium arsenide can be found in ref. 30 ; for simplicity we have assumed background permittivity of InAs to be unity. We have modeled bismuth iron garnet with a fixed dielectric permittivity ε mo =6.25, that is, we have neglected the losses and dispersion in this material, assuming that dispersion and dissipation in metal have a more significant role. The off-diagonal term of permittivity tensor for bismuth iron garnet saturates at α sat =0.06 for B =150 mT (ref. 23 ). The dependence of α on magnetization can be estimated from experimental data on Faraday rotation in bulk bismuth iron garnet with material magnetization. In particular, in a first order approximation we have modeled this response as α = α sat tanh[ ηB ( ρ )], where 1/ η ≃ 30 mT is a phenomenological coefficient determined from experiment [23] . How to cite this article: Davoyan, A. and Engheta, N. Electrically controlled one-way photon flow in plasmonic nanostructures. Nat. Commun. 6:5250 doi: 10.1038/ncomms6250 (2014).